The adipokine Retnla modulates cholesterol homeostasis in hyperlipidemic mice Hyperlipidemia is a well-recognized risk factor for atherosclerosis and can be regulated by adipokines. Expression of the adipokine resistin-like molecule alpha (Retnla) is regulated by food intake; whether Retnla has a role in the pathogenesis of hyperlipidemia and atherosclerosis is unknown. Here we report that Retnla has a cholesterol-lowering effect and protects against atherosclerosis in low-density lipoprotein receptor-deficient mice. On a high-fat diet, Retnla deficiency promotes hypercholesterolaemia and atherosclerosis, whereas Retnla overexpression reverses these effects and improves the serum lipoprotein profile, with decreased cholesterol in the very low-density lipoprotein fraction concomitant with reduced serum apolipoprotein B levels. We show that Retnla upregulates cholesterol-7-α-hydroxylase, a key hepatic enzyme in the cholesterol catabolic pathway, through induction of its transcriptional activator liver receptor homologue-1, leading to increased excretion of cholesterol in the form of bile acids. These findings define Retnla as a novel therapeutic target for treating hypercholesterolaemia and atherosclerosis. Atherosclerosis remains one of the leading causes of morbidity and mortality worldwide [1] . The progression of atherosclerosis is affected by various adipokines, cytokines produced primarily by adipose tissue [2] , [3] . Most adipokines, including leptin [4] , tumor necrosis factor-α (TNF-α) [5] , interleukin (IL)-18 (ref. 6 ) and resistin [7] , have been shown to promote atherosclerosis. Conversely, adiponectin is considered an adipokine that protects against atherosclerosis [8] . The ‘resistin-like molecules (Relm)’ family, also known as ‘found in inflammatory zone’ proteins, is a group of small cysteine-rich secreted proteins that are highly conserved in mammals, including humans and mice [9] . Resistin-like molecule alpha (Retnla)/Relm-α/FIZZ1, Retnlb/Relm-β/FIZZ2, Retn/Resistin/FIZZ3 and Retnlg/Relm-γ/FIZZ4 are all members of this gene family [9] . The mouse genome contains genes encoding for all members of the gene family, but in human, only two members, RETNLB and resistin have been identified [9] . Retnla, adipokine, was initially found in allergic lung inflammation [10] . Its expression has been reported in lung, spleen, heart and mammary glands, as well as in white adipose tissue (WAT) [10] , [11] , [12] , and is highly inducible in epithelial cells, macrophages and eosinophils after inflammatory stimulations associated with parasites infection, allergy and tissue injury [10] , [13] , [14] . Exposure to the T helper (Th)2 cytokines IL-4 and IL-13 or environments involved in Th2 immune responses increased the expression of Retnla, identifying Retnla as a hallmark signature gene for alternatively activated macrophages [14] , [15] , [16] . Thus, Retnla has been implicated most in association with inflammation. Recent evidence has revealed possible roles of Retnla in metabolic regulation. For example, Retnla inhibited differentiation of adipocytes [17] and was downregulated in food-restricted mice [18] , [19] , lactating mice [20] and leptin receptor −/− ( db / db ) mice, a model of obesity and type 2 diabetes [21] . Nevertheless, the function of Retnla in metabolic regulation is yet to be defined. Hypercholesterolaemia, a condition of high cholesterol levels in blood, is a major risk factor of atherosclerosis [22] , [23] . Elevated levels of circulating cholesterol reflect increased levels of circulating lipoprotein, cholesterol-carrier molecules that are assembled and secreted by the liver [24] , [25] . In the blood, there are three types of lipoproteins, very low-density lipoprotein (VLDL) and its metabolite low-density lipoprotein (LDL), as well as high-density lipoprotein (HDL). VLDL and LDL carry most of the circulating cholesterols and have proatherogenic effects; they contribute to the formation of atherosclerotic lesions by transporting and depositing cholesterols into arterial vessel walls [23] , [26] . HDL has anti-atherogenic effects through reverse cholesterol transport [23] . Thus, high levels of serum VLDL and LDL cholesterols and low levels of HDL cholesterol are primary risk factors for atherosclerosis. Intensive efforts are underway in the search for optimized therapies to regulate cholesterol and lipoprotein levels. Bile acids, the end-products of hepatic cholesterol catabolism, are important for eliminating excess cholesterols from the body [27] . A severely reduced rate of bile acid synthesis is associated with hepatic accumulation of cholesterol, which leads to secretion of cholesterol-rich lipoproteins from the liver and the build-up of atherosclerotic plaques in the arteries [28] . Therefore, the removal of excessive cholesterols by bile acid formation is a promising therapeutic target for hypercholesterolaemia and atherosclerosis. Two different pathways have been identified for cholesterol conversion of bile acid: the classical pathway and the alternative pathway [29] . The classical pathway accounts for the majority of total bile acid synthesis and is mediated by cholesterol-7-α-hydroxylase (CYP7A1), the first and rate-limiting enzyme of the pathway [30] . Both gain- and loss-of-function studies have demonstrated that CYP7A1 plays an important role in the pathogenesis of hypercholesterolaemia and atherosclerosis [31] , [32] , [33] . For example, studies by Miyake et al . [31] and Li et al . [32] demonstrated that transgenic expression of CYP7A1 in mice leads to large decreases in VLDL and LDL cholesterol levels in the plasma and protects from gallstone formation and atherosclerosis during exposure to a high-fat, high-cholesterol (HFHC) diet. Patients with CYP7A1 deficiency have been shown to develop elevated plasma LDL cholesterol levels and hepatic cholesterol contents, gallstones and premature atherosclerosis [33] . Considering the beneficial or detrimental effects of adipokines in the processes of atherosclerosis, we hypothesized that Retnla may play a critical role in atherosclerosis caused by a metabolic defect, especially hyperlipidemia. To investigate the precise role of Retnla in hyperlipidemia-induced atherosclerosis, we used LDL receptor-deficient ( Ldlr −/− ) mice that either overexpress or lack Retnla. We found that Retnla is a critical adipokine for regulating increased serum concentrations of cholesterol under hyperlipidemic conditions in these two different rodent models. Our work shows that Retnla is a key regulator of the cholesterol catabolic processes that produces bile acid in response to increased serum cholesterol through liver receptor homologue-1 (Lrh-1)-mediated induction of Cyp7a1 expression under hyperlipidemic states. Such features allow Retnla to efficiently control atherosclerosis formation. Retnla is induced under a hyperlipidemic state To address the relationship between Retnla and hyperlipidemia, we initially examined the effect of a high-fat diet (HFD) on the expression levels of Retnla in WAT and whole blood from wild-type (WT) C57BL/6J mice. Consistent with a previous report [19] , Retnla expression in adipose tissue was limited to the stromal vascular fraction (SVF) ( Fig. 1a ). Using immunofluorescence staining, we confirmed that Retnla is expressed in the stroma of WAT ( Fig. 1b ). Surprisingly, we found that Retnla levels were significantly increased in the SVF from WT C57BL/6J mice fed a HFD for 4 weeks when compared with normolipidemic controls ( Fig. 1a,c ). Serum levels of Retnla were also significantly increased in WT C57BL/6J mice after 4 weeks of HFD feeding when compared with normolipidemic controls ( Fig. 1d ). These data suggest that Retnla levels in SVF in adipose tissues and blood are associated with hyperlipidemia in vivo and were confirmed using two different mouse models of hyperlipidemia, Ldlr −/− and ob / ob mice, which exhibit mild hyperlipidemia on a standard diet (SD) but develop severe hyperlipidemia on a HFD [34] , [35] . Although the serum Retnla levels were similar in Ldlr −/− mice and control animals fed a SD, they were significantly higher in Ldlr −/− mice than control animals after 4 weeks of HFD feeding ( Fig. 1e,f ). Despite receiving a SD, ob / ob mice also showed significantly higher serum Retnla levels than control animals ( Fig. 1g ). These data provide further support for the relationship between serum Retnla levels and hyperlipidemia. 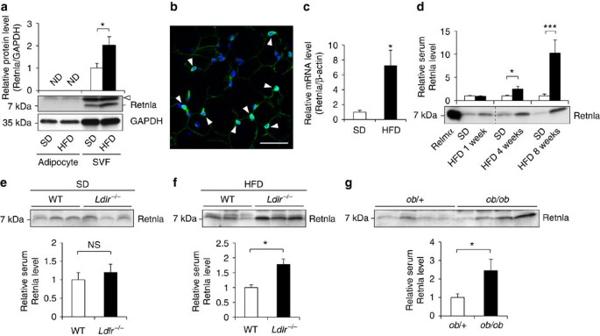Figure 1: Hyperlipidemia induces Retnla expression in the SVF of adipose tissue and serum. (a) Representative immunoblot analysis (bottom) and quantification (top) of Retnla expression in the SVF and adipocytes from epididymal fat of 12-week-old C57BL/6J mice fed SD or HFD for 4 weeks (n=5 per group). Glyceraldehyde-3-phosphate dehydrogenase (GAPDH) was also analysed as a loading control. Open arrowhead indicates a nonspecific band. ND, not detected. (b) Immunofluorescence staining of Retnla and nuclear counterstaining with 4',6-diamidino-2-phenylindole dihydrochloride in epididymal fat of C57BL/6J mice. Immunoreactivities of Retnla (arrowhead) are shown. Scale bar, 50 μm. (c) qRT–PCR analysis of the Retnla gene in the SVF of C57BL/6J mice fed a SD or HFD for 4 weeks (n=5 per group). (d) Representative immunoblot analysis (bottom) and quantification (top) of Retnla levels in serum from C57BL/6J mice fed a HFD for the indicated period (n=5 per group). rRelmα (2.5 ng) was used as a positive control. Dashed line indicates that lanes were run on the same gel but were noncontiguous. (e,f) Representative immunoblot analysis (top) and quantification (bottom) of Retnla in serum from male 12-week-old WT andLdlr−/−mice fed (e) a SD or (f) a HFD for 4 weeks (n=7–8 per group). NS, not significant. (g) Representative immunoblot analysis (top) and quantification (bottom) of Retnla in serum from maleob/obandob/+ mice at 8 weeks of age (n=5 per group). Data are presented as mean±s.e.m. according to the Mann–WhitneyU-test; *P<0.05; ***P<0.005. Full scan images of immunoblots are shown inSupplementary Fig. 1. Figure 1: Hyperlipidemia induces Retnla expression in the SVF of adipose tissue and serum. ( a ) Representative immunoblot analysis (bottom) and quantification (top) of Retnla expression in the SVF and adipocytes from epididymal fat of 12-week-old C57BL/6J mice fed SD or HFD for 4 weeks ( n =5 per group). Glyceraldehyde-3-phosphate dehydrogenase (GAPDH) was also analysed as a loading control. Open arrowhead indicates a nonspecific band. ND, not detected. ( b ) Immunofluorescence staining of Retnla and nuclear counterstaining with 4',6-diamidino-2-phenylindole dihydrochloride in epididymal fat of C57BL/6J mice. Immunoreactivities of Retnla (arrowhead) are shown. Scale bar, 50 μm. ( c ) qRT–PCR analysis of the Retnla gene in the SVF of C57BL/6J mice fed a SD or HFD for 4 weeks ( n =5 per group). ( d ) Representative immunoblot analysis (bottom) and quantification (top) of Retnla levels in serum from C57BL/6J mice fed a HFD for the indicated period ( n =5 per group). rRelmα (2.5 ng) was used as a positive control. Dashed line indicates that lanes were run on the same gel but were noncontiguous. ( e , f ) Representative immunoblot analysis (top) and quantification (bottom) of Retnla in serum from male 12-week-old WT and Ldlr −/− mice fed ( e ) a SD or ( f ) a HFD for 4 weeks ( n =7–8 per group). NS, not significant. ( g ) Representative immunoblot analysis (top) and quantification (bottom) of Retnla in serum from male ob / ob and ob /+ mice at 8 weeks of age ( n =5 per group). Data are presented as mean±s.e.m. according to the Mann–Whitney U -test; * P< 0.05; *** P< 0.005. Full scan images of immunoblots are shown in Supplementary Fig. 1 . Full size image Retnla deficiency increases serum cholesterol and atherosclerosis To define the role of Retnla in vivo , we generated Retnla -deficient ( Retnla −/− ) mice using a targeting vector in which the neo cassette was introduced into the coding region of the Retnla gene ( Fig. 2a ). Germline transmission of the mutant allele was confirmed by Southern blot analysis ( Fig. 2b ). Genotypic distributions in the offspring followed a Mendelian inheritance pattern, and all knockout mice used in the present study were normal in appearance. Genetic ablation of Retnla was confirmed by assessing serum levels of Retnla in WT and Retnla −/− mice ( Fig. 2c ). To examine whether there was any compensatory change in expression of other Relm family members in Retnla −/− mice, messenger RNA (mRNA) levels of Retnlb, resistin and Retnlg were determined by quantitative real-time PCR (qRT–PCR) in WAT ( Supplementary Fig. 2 ). Loss of Retnla expression did not alter WAT mRNA levels of other Relm family members in mice on a SD or HFD ( Supplementary Fig. 2 ). In addition, loss of Retnla expression did not result in compensatory changes in serum levels of adiponectin, a unique adipokine with anti-inflammatory and anti-atherogenic effects [3] , under either normolipidemic or hyperlipidemic states ( Supplementary Fig. 3 ). 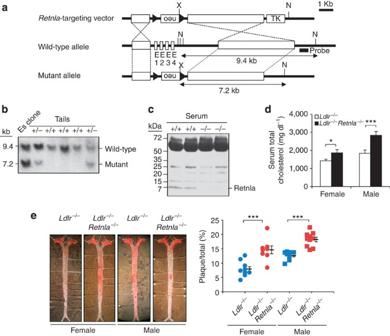Figure 2: Retnla deficiency promotes hypercholesterolaemia and atherosclerosis inLdlr−/−mice. (a) Targeting vector for generatingRetnla-deficient mice (Retnla−/−). (b) Southern blot analysis of genomic DNA from mice with the indicated genotypes. DNA was digested withNcoI (N) andXhoI (X) for genotyping as indicated ina. Hybridized probes are indicated ina. (c) Immunoblot analysis of Retnla in serum fromRetnla−/−and WT mice. (d) Serum total cholesterol levels inLdlr−/−Retnla−/−andLdlr−/−mice fed a HFD for 18 weeks (n=8–10 in each group). (e)En faceview of Oil red O-stained lesions in aortas from the same mice as ind. Left: illustrative stains; right: measurements of atherosclerotic lesion size in aortas from individual mice. Data are presented as mean±s.e.m. according to the Mann–WhitneyU-test; *P<0.05; ***P<0.005. Figure 2: Retnla deficiency promotes hypercholesterolaemia and atherosclerosis in Ldlr −/− mice. ( a ) Targeting vector for generating Retnla -deficient mice ( Retnla −/− ). ( b ) Southern blot analysis of genomic DNA from mice with the indicated genotypes. DNA was digested with Nco I (N) and Xho I (X) for genotyping as indicated in a . Hybridized probes are indicated in a . ( c ) Immunoblot analysis of Retnla in serum from Retnla −/− and WT mice. ( d ) Serum total cholesterol levels in Ldlr −/− Retnla −/− and Ldlr −/− mice fed a HFD for 18 weeks ( n =8–10 in each group). ( e ) En face view of Oil red O-stained lesions in aortas from the same mice as in d . Left: illustrative stains; right: measurements of atherosclerotic lesion size in aortas from individual mice. Data are presented as mean±s.e.m. according to the Mann–Whitney U -test; * P< 0.05; *** P< 0.005. Full size image As Retnla expression was induced during hyperlipidemic conditions, we aimed to determine the effects of Retnla deficiency on hyperlipidemia-induced atherosclerosis. We cross-bred Retnla −/− mice with hyperlipidemia- and atherosclerosis-susceptible Ldlr -deficient ( Ldlr −/− ) mice to produce Retnla and Ldlr double mutant ( Ldlr −/− Retnla −/− ) mice ( Supplementary Fig. 4 ). Age- and sex-matched Ldlr −/− Retnla −/− and Ldlr −/− mice were fed a HFD for 18 weeks. Food intake was similar between both genotypes fed the HFD ( Supplementary Fig. 5a ). During the HFD feeding period, body and liver weights were significantly higher in Ldlr −/− Retnla −/− male mice compared with male Ldlr −/− mice, with an increase in fat pad weight ( P =0.60, Mann–Whitney U -test) ( Supplementary Fig. 5b–d ). However, in female mice, there were no significant differences in the weights for body, liver or fat pads between Ldlr −/− Retnla −/− and Ldlr −/− animals ( Supplementary Fig. 5b–d ). Despite the difference between male and female mice, serum total cholesterol levels showed significant increases by ~23 and 30%, respectively, in Ldlr −/− Retnla −/− female and male mice ( Fig. 2d ). The atherosclerotic lesion area determined by en face analyses of total aortic surfaces increased ~2.2-fold and 1.4-fold in Ldlr −/− Retnla −/− female and male mice, respectively ( Fig. 2e ). These results indicate that Retnla has a protective role in HFD-induced hypercholesterolaemia and atherosclerosis. Retnla deficiency promotes macrophage accumulation in atheroma Given that Retnla is an alternatively activated macrophage-inducible gene [15] , [16] that modulates immune responses in inflammatory diseases [13] , [18] , [36] , [37] , and that atherosclerosis can be considered both a lipid metabolism disorder and a chronic inflammatory disease [23] , we examined whether Retnla deficiency also influences inflammatory plaque phenotypes. Consistent with the increased en face plaque area, aortic root lesions were also increased in Ldlr −/− Retnla −/− mice compared with Ldlr −/− mice ( Fig. 3a,b , top panel). Immunofluorescence staining revealed more abundant macrophages in the lesions of Ldlr −/− Retnla −/− mice compared with Ldlr −/− mice ( Fig. 3a,b , second panel from the top). We also observed increased cell death in the atherosclerotic lesions of Ldlr −/− Retnla −/− mice compared with those of Ldlr −/− mice by measuring the necrotic core in lesions from the two genotypes ( Fig. 3a,b , third panel from the top). The collagen content was similar in the lesions of both groups of mice ( Fig. 3a,b , bottom panel). In the atherosclerotic plaque lesions, there are two distinct macrophage subtypes: the proinflammatory macrophages, also known as classically activated (M1) macrophages, and anti-inflammatory macrophages, also known as alternatively activated (M2) macrophages [38] . Given that differentiation into M1 and M2 subsets of macrophage is critically related to atherosclerosis progression [38] , we tested the effect of Retnla deficiency on macrophage types within plaques by analysing M1- and M2-associated genes by qRT–PCR of RNA extracted from aortas of Ldlr −/− Retnla −/− and Ldlr −/− mice. Among the M1-associated genes such as Il6, Mcp1, Ifnγ and Cd16, Il6 expression was increased by Retnla deficiency, but the difference was not significant ( Supplementary Fig. 6a ). Expression of the M2-associated genes, such as Mgl1, Arg1, Ym1 and Cd36, were also not significantly changed by Retnla deficiency ( Supplementary Fig. 6b ). To further examine the effects of Retnla deficiency on macrophage phenotypes in vitro , we analysed the M1/M2 markers in peritoneal macrophages from Retnla −/− and WT mice using well-established M1 (lipopolysaccharide; LPS) or M2 (IL-4) polarizing agents [39] . Expression of M1/M2 genes in Retnla −/− microphages did not differ from those of WT macrophages in either the absence or presence of LPS or IL-4 ( Supplementary Fig. 6c,d ). Taken together, these results suggest that Retnla deficiency contributes to acceleration of atherogenesis with no significant changes in macrophage differentiation. 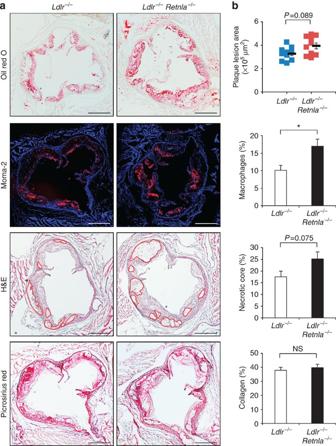Figure 3: Retnla deficiency affects aortic lesion composition inLdlr−/−mice. (a) From the top panel to the bottom panel, representative cross-sections of Oil red O staining for atherosclerotic lesions, immunostaining for monocyte and macrophage antibody-2 (Moma-2), hematoxylin and eosin (H&E) staining for necrotic core detection and picrosirius red staining of collagen (in red) on aortic sinus fromLdlr−/−Retnla−/−andLdlr−/−mice fed a HFD for 18 weeks (n=13 forLdlr−/−male mice,n=14 forLdlr−/−/Retnla-Tg male mice). Scale bar, 400 μm. The atherosclerotic lesion size was measured in aortas from individual mice. (b) Quantification of lipid, macrophage, necrotic core and collagen content in atherosclerotic lesions in the two groups. Individual symbols in Oil red O staining represent the lesion area measurements from an individual mouse. The macrophage content, necrotic core and collagen content were defined as mean percentage relative to mean total plaque area using 2–3 consecutive sections per mouse. Red lines in H&E staining show the boundaries of the developing necrotic core. NS, not significant. Data are presented as mean±s.e.m. according to Mann–WhitneyU-test; *P<0.05. Figure 3: Retnla deficiency affects aortic lesion composition in Ldlr −/− mice. ( a ) From the top panel to the bottom panel, representative cross-sections of Oil red O staining for atherosclerotic lesions, immunostaining for monocyte and macrophage antibody-2 (Moma-2), hematoxylin and eosin (H&E) staining for necrotic core detection and picrosirius red staining of collagen (in red) on aortic sinus from Ldlr −/− Retnla −/− and Ldlr −/− mice fed a HFD for 18 weeks ( n =13 for Ldlr −/− male mice, n =14 for Ldlr −/− / Retnla -Tg male mice). Scale bar, 400 μm. The atherosclerotic lesion size was measured in aortas from individual mice. ( b ) Quantification of lipid, macrophage, necrotic core and collagen content in atherosclerotic lesions in the two groups. Individual symbols in Oil red O staining represent the lesion area measurements from an individual mouse. The macrophage content, necrotic core and collagen content were defined as mean percentage relative to mean total plaque area using 2–3 consecutive sections per mouse. Red lines in H&E staining show the boundaries of the developing necrotic core. NS, not significant. Data are presented as mean±s.e.m. according to Mann–Whitney U -test; * P< 0.05. Full size image Retnla reduces serum cholesterol and ameliorates atherosclerosis To test whether increased serum Retnla alleviates hypercholesterolaemia and atherosclerosis in vivo , we generated Retnla -overexpressing ( Retnla -Tg) mice. Confirmation of overexpression was determined by assessing serum Retnla levels in WT and Retnla -Tg mice ( Supplementary Fig. 7a,b ). Retnla -Tg mice were healthy and fertile. The expression of Retnlg was slightly decreased in WAT from Retnla -Tg mice; however, the expressions of other Relm family isoforms were not changed ( Supplementary Fig. 8 ). Serum adiponectin levels were not different between the two genotypes ( Supplementary Fig. 9 ). Since C57BL/6J background Retnla -Tg mice do not develop measureable atherosclerotic plaque lesions on a HFHC diet ( Supplementary Fig. 10 ), we further cross-bred Retnla -Tg mice with Ldlr −/− mice to generate Retnla -overexpressing Ldlr −/− ( Ldlr −/− / Retnla -Tg) mice ( Supplementary Fig. 11 ), and we subjected age- and sex-matched Ldlr −/− / Retnla -Tg and Ldlr −/− mice to a HFD for 10 and 28 weeks. At 10 weeks, the total en face aortic lesion area was reduced in Ldlr −/− / Retnla -Tg female and male mice, but the statistical difference was not significant ( Supplementary Fig. 12 ). After 28 weeks on the diet, the total en face aortic lesion area was reduced by ~19 and 29% in Ldlr −/− / Retnla -Tg female and male mice, respectively ( Fig. 4a ). Aortic root lesions were also decreased by ~21 and 15% in Ldlr −/− /Retnla -Tg female and male mice, respectively ( Fig. 4b ). Food intake and weights for body, liver and epididymal fat pad were similar between the genotypes fed the HFD for 28 weeks ( Supplementary Fig. 13a–d ). Similar reductions in en face lesion areas were observed in Ldlr −/− / Retnla -Tg female and male mice generated by cross-breeding Ldlr −/− mice with another Retnla -Tg line (the 0011 mouse line) (~30 and 25% in female and male mice, respectively) ( Supplementary Fig. 14a ). Total serum cholesterol levels were also decreased by ~29 and 19% in Ldlr −/− / Retnla -Tg female and male mice, respectively, fed a HFD for 28 weeks ( Fig. 4c ). A similar reduction in serum total cholesterol levels was observed in Ldlr −/− / Retnla -Tg female and male mice generated by cross-breeding Ldlr −/− mice with the 0011 Retnla -Tg line (~31 and 15% in female and male mice, respectively) ( Supplementary Fig. 14b ). In addition, fast protein lipid chromatography (FPLC) analysis of serum lipoprotein profiles revealed that the decreased serum cholesterol levels in Ldlr −/− / Retnla -Tg mice were mostly caused by the dramatic reduction in the cholesterol content of VLDL, the serum lipoprotein associated with an increased risk of atherosclerosis in mice [26] (~58 and 47% in female and male mice, respectively) ( Fig. 4d ). Consistent with these data, the content of apolipoprotein (apo) B, the key structural protein in the formation of VLDL [40] , in the VLDL fractions was markedly decreased in Ldlr −/− / Retnla -Tg mice compared with Ldlr −/− mice ( Fig. 4d , see inset ). These results were also consistent with the decreased apoB content in whole serum ( Fig. 4e ; Supplementary Fig. 15a,b ). These favourable responses observed in Ldlr −/− / Retnla -Tg mice further support a protective role of Retnla in hypercholesterolaemia and atherosclerosis in vivo . 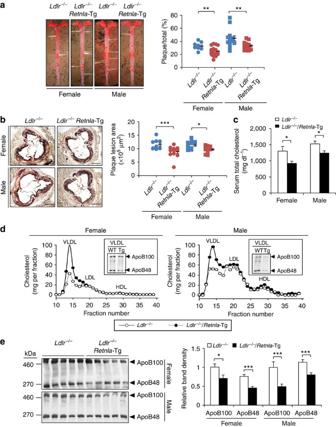Figure 4: Overexpression of Retnla protects against atherosclerosis and reduces the levels of serum VLDL cholesterol inLdlr−/−mice. (a,b) Oil red O-stained aortic sinuses (a) and en faceaortas (b) fromLdlr−/−/Retnla-Tg andLdlr−/−mice fed a HFD for 28 weeks. Left: illustrative stains; right: measurements of atherosclerotic lesion size in aortas from individual mice (n=9 forLdlr−/−female mice,n=16 forLdlr−/−/Retnla-Tg female mice,n=13 forLdlr−/−male mice,n=14 forLdlr−/−/Retnla-Tg male mice). Scale bar, 400 μm. (c) Total cholesterol levels in serum from the same mice as ina,b. (d) Representative FPLC analysis for serum lipoprotein distribution inLdlr−/−/Retnla-Tg andLdlr−/−control mice. Pooled serum samples (200 μl) from the same mice as inaandbwere used for FPLC analysis. Boxes in the graph show the immunoblot analysis of apoB100 and apoB48 contained within the VLDL top fraction. (e) Representative immunoblot analysis for apoB100 and apoB48 in 1 μl serum from the same mice as ina,b. Quantification by densitometry is to the right of the immunoblot. Data are presented as mean±s.e.m. according to the Mann–WhitneyU-test; *P<0.05; **P<0.01; ***P<0.005. Figure 4: Overexpression of Retnla protects against atherosclerosis and reduces the levels of serum VLDL cholesterol in Ldlr −/− mice. ( a , b ) Oil red O-stained aortic sinuses ( a ) and e n face aortas ( b ) from Ldlr −/− / Retnla -Tg and Ldlr −/− mice fed a HFD for 28 weeks. Left: illustrative stains; right: measurements of atherosclerotic lesion size in aortas from individual mice ( n =9 for Ldlr −/− female mice, n =16 for Ldlr −/− / Retnla -Tg female mice, n =13 for Ldlr −/− male mice, n =14 for Ldlr −/− / Retnla -Tg male mice). Scale bar, 400 μm. ( c ) Total cholesterol levels in serum from the same mice as in a , b . ( d ) Representative FPLC analysis for serum lipoprotein distribution in Ldlr −/− / Retnla -Tg and Ldlr −/− control mice. Pooled serum samples (200 μl) from the same mice as in a and b were used for FPLC analysis. Boxes in the graph show the immunoblot analysis of apoB100 and apoB48 contained within the VLDL top fraction. ( e ) Representative immunoblot analysis for apoB100 and apoB48 in 1 μl serum from the same mice as in a , b . Quantification by densitometry is to the right of the immunoblot. Data are presented as mean±s.e.m. according to the Mann–Whitney U -test; * P< 0.05; ** P< 0.01; *** P< 0.005. Full size image Retnla induces Lrh-1-mediated Cyp7a1 gene expression To explore the molecular mechanisms underlying the cholesterol-lowering effects of Retnla under hyperlipidemic conditions, we subjected age- and sex-matched Retnla -Tg and control mice to a HFD for 1, 2 and 4 weeks. As expected, serum cholesterol levels were lower in Retnla -Tg mice compared with HFD-fed WT mice ( Fig. 5a ) but were similar between both genotypes when fed a SD ( Supplementary Fig. 7c ). We analysed the hepatic gene expression profiles related to cholesterol metabolism, including catabolism, biosynthesis and transport, using a microarray approach. Resultant expression profiling was shown by fold change ( Supplementary Table 1 ). The most significant change in Retnla -Tg mice was an upregulation of Cyp7a1, the rate-limiting enzyme in the conversion of cholesterol into bile acids [29] . Gene expression profiling from the GeneChip assay was confirmed by qRT–PCR ( Fig. 5b ; Supplementary Table 1 ). Although Sterol 12α-hydroxylase (Cyp8b1), a downstream enzyme of bile acid synthesis [29] , showed no significant differences in the microarray, qRT–PCR analysis revealed that it, too, was upregulated in Retnla -Tg mice ( Fig. 5b ). There were no significant differences in other tested enzymes, oxysterol 7α-hydroxylase (Cyp7b1) or sterol 27-hydroxylase (Cyp27a1), which are related to the alternative pathway of bile acid synthesis [29] ( Supplementary Table 1 ). In addition, the expression levels of other genes involved in cholesterol biosynthesis and transport processes were not altered by Retnla overexpression ( Supplementary Table 1 ). Consistent with these data, an increase in the Cyp7a1 mRNA level accompanied by a decrease in the serum total cholesterol levels was observed in Ldlr −/− / Retnla -Tg mice compared with controls ( Supplementary Fig. 16a,b ). Thus, it appears that the enhanced cholesterol catabolism mediated primarily by Cyp7a1 and Cyp8b1 is responsible for the cholesterol-lowering effect of Retnla. 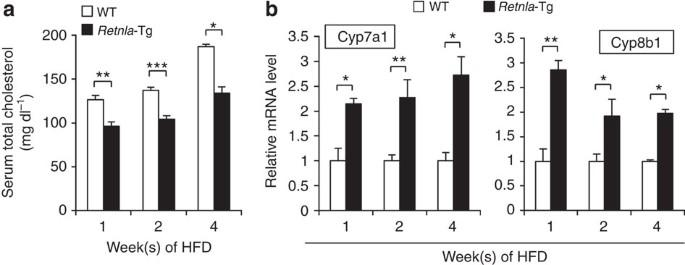Figure 5: Overexpression of Retnla induces the expressions of Cyp7a1 and Cyp8b1 in mice livers. (a) Total serum cholesterol levels were measured in WT andRetnla-Tg mice fed a HFD for the indicated periods (n=4–7 per group). (b) The mRNA levels of Cyp7a1 and Cyp8b1 were determined by qRT–PCR analysis of RNA from the livers of the same mice as ina. Data are presented as mean±s.e.m. according to the Mann–WhitneyU-test; *P<0.05; **P<0.01; ***P<0.005. Figure 5: Overexpression of Retnla induces the expressions of Cyp7a1 and Cyp8b1 in mice livers. ( a ) Total serum cholesterol levels were measured in WT and Retnla -Tg mice fed a HFD for the indicated periods ( n =4–7 per group). ( b ) The mRNA levels of Cyp7a1 and Cyp8b1 were determined by qRT–PCR analysis of RNA from the livers of the same mice as in a . Data are presented as mean±s.e.m. according to the Mann–Whitney U -test; * P< 0.05; ** P< 0.01; *** P< 0.005. Full size image To confirm the findings of the hepatic mRNA profiling in vivo , we examined the effect of Retnla in AML-12 cells, a mouse hepatocyte cell line. Treatment of AML-12 cells with recombinant mouse Retnla protein (rRelmα) caused increases in Cyp7a1 and Cyp8b1 mRNA expression of ~2.5-fold and 3.5-fold, respectively, after 6 h of treatment ( Fig. 6a ). To identify the signalling pathway that mediates upregulation of the Cyp7a1 gene by Retnla, we studied the effect of Retnla on the expression of several key transcription factors involved in the regulation of the Cyp7a1 gene, including Lrh-1, farnesoid X receptor, small heterodimer partner, liver X receptor α, hepatocyte nuclear factor-4α, albumin D-site-binding protein 1, peroxisome proliferator-activated receptor-α, sterol regulatory element binding protein-1c and sterol regulatory element binding protein 2 (refs 29 , 41 , 42 ). After 3 h of treatment, rRelmα caused induction of Lrh-1 mRNA expression; the expression level was maintained at an approximately twofold level until 12 h ( Fig. 6a ). However, we did not observe any effect of Retnla on the mRNA expression of genes other than Lrh-1 ( Fig. 6a ; Supplementary Fig. 17a–d ). A similar induction of Lrh-1 mRNA expression was observed in Retnla -Tg mice compared with HFD-fed control animals ( Supplementary Fig. 18 ), despite no significant differences being observed in the microarray. 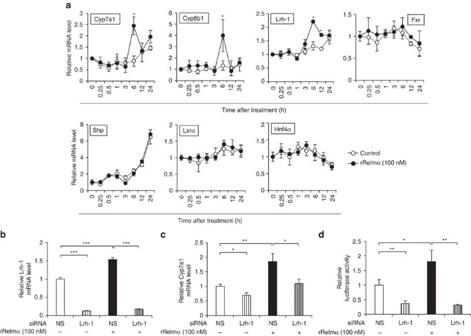Figure 6: Retnla increases Lrh-1-mediated Cyp7a1 expression in AML-12 hepatocytes. (a) mRNA levels of Cyp7a1, Cyp8b1, Lrh-1, farnesoid X receptor (Fxr), small heterodimer partner (Shp), liver X receptor α (Lxrα) and hepatocyte nuclear factor-4α (Hnf4α) were determined by qRT–PCR analysis of RNA from AML-12 cells treated with rRelmα (100 nM) for the indicated time period. (b,c) The mRNA levels of (b) Lrh-1 and (c) Cyp7a1 were determined by qRT–PCR analysis of RNA from AML-12 cells transfected with siRNA against Lrh-1 or non-silencing siRNA in absence or presence of rRelmα. (d) Mouse Cyp7a1 promoter activity in response to rRelmα treatment was measured in AML-12 cells transfected with Lrh-1 or non-silencing siRNA. Data are presented as mean±s.e.m. from two independent experiments in triplicate (a), three independent experiments with at least four replicates (b,c) or three independent experiments in triplicate (d). Student’st-test; *P<0.05; **P<0.01; ***P<0.005. Figure 6: Retnla increases Lrh-1-mediated Cyp7a1 expression in AML-12 hepatocytes. ( a ) mRNA levels of Cyp7a1, Cyp8b1, Lrh-1, farnesoid X receptor (Fxr), small heterodimer partner (Shp), liver X receptor α (Lxrα) and hepatocyte nuclear factor-4α (Hnf4α) were determined by qRT–PCR analysis of RNA from AML-12 cells treated with rRelmα (100 nM) for the indicated time period. ( b , c ) The mRNA levels of ( b ) Lrh-1 and ( c ) Cyp7a1 were determined by qRT–PCR analysis of RNA from AML-12 cells transfected with siRNA against Lrh-1 or non-silencing siRNA in absence or presence of rRelmα. ( d ) Mouse Cyp7a1 promoter activity in response to rRelmα treatment was measured in AML-12 cells transfected with Lrh-1 or non-silencing siRNA. Data are presented as mean±s.e.m. from two independent experiments in triplicate ( a ), three independent experiments with at least four replicates ( b , c ) or three independent experiments in triplicate ( d ). Student’s t -test; * P< 0.05; ** P< 0.01; *** P< 0.005. Full size image To test whether Cyp7a1 induction by Retnla requires Lrh-1, Lrh-1 was knocked down in AML-12 cells using small interfering RNA (siRNA). Transfection of AML-12 cells with siRNA targeting murine Lrh-1 resulted in a nearly complete loss of Lrh-1 mRNA expression relative to that in cells transfected with non-silencing siRNA ( Fig. 6b ). Importantly, rRelmα treatment induced Lrh-1 mRNA expression, but the induction was nearly eliminated by Lrh-1 knockdown ( Fig. 6b ). Lrh-1 knockdown also repressed Cyp7a1 mRNA levels by ~30% and abolished Cyp7a1 induction by rRelmα treatment, reaching a level similar to that observed in cells transfected with non-silencing siRNA in the absence of rRelmα ( Fig. 6c ). Given that Lrh-1 acts as a positive regulator of Cyp7a1 transcription [41] , [42] , we performed luciferase reporter assays to determine whether Retnla-induced Cyp7a1 expression is mediated through the transactivation of the Cyp7a1 promoter by Lrh-1. Lrh-1 knockdown led to ~70% suppression of Cyp7a1 promoter activity, while rRelmα treatment showed an increase of ~70% on Cyp7a1 promoter activity ( Fig. 6d ). Simultaneous Lrh-1 siRNA and rRelmα treatment, however, failed to induce Cyp7a1 promoter activity ( Fig. 6d ). These data demonstrate that Lrh-1 is essential for Retnla-induced Cyp7a1 expression. Although the receptor for Retnla remains unknown, our results showed that Retnla could be involved in hepatic signalling in a paracrine or endocrine manner. Consistent with a previous report [12] , Retnla was not detected in the liver from WT C57BL/6J mice ( Supplementary Fig. 19a ), indicating endocrine action of Retnla signalling in the liver. We tried to indirectly demonstrate the existence of the Retnla receptor by performing a Retnla-binding assay on AML-12 cells. Alexa Fluor-labelled rRelmα was localized on the outer margin of the plasma membrane of these cells ( Supplementary Fig. 19b , top). In addition, excessive treatment with unlabelled rRelmα blocked the binding of Alexa Fluor-labelled rRelmα ( Supplementary Fig. 19b , middle and bottom), suggesting the presence of a receptor for Retnla in hepatocytes. Retnla increases bile acid excretion Key hepatic enzymes such as Cyp7a1 and Cyp8b1 tightly regulate the bile acid biosynthetic pathway [29] ; therefore, we tested whether Retnla affected hepatic cholesterol homeostasis by regulating bile acid production. The bile acid pool was increased in Retnla -Tg mice compared with WT controls, but the difference was not statistically significant ( Supplementary Fig. 20 ). Nevertheless, the hepatic content of bile acid increased by ~17% in Retnla -Tg mice fed a HFD for 2 weeks ( Fig. 7a ), accompanied by an ~17% reduction in hepatic cholesterol levels ( Fig. 7b ). Moreover, the faecal excretion of bile acid and cholesterol was higher in Retnla -Tg mice (32 and 23%, respectively) ( Fig. 7c,d ). Similarly, Ldlr −/− /Retnla -Tg mice also showed increases of ~19%, 27% and 26% in hepatic and faecal bile acid content and faecal cholesterol excretion, respectively ( Fig. 7e,g,h ) and a decrease of ~21% in hepatic cholesterol content ( Fig. 7f ). In addition, serum bile acid levels were decreased by ~62% in Ldlr −/− /Retnla -Tg mice ( Supplementary Fig. 21 ). Collectively, these results indicate that Retnla ameliorates HFD-induced hypercholesterolaemia and atherosclerosis by promoting the conversion of cholesterol into bile acid and mediating its subsequent faecal excretion via Lrh-1-mediated Cyp7a1 regulation ( Fig. 8 ). 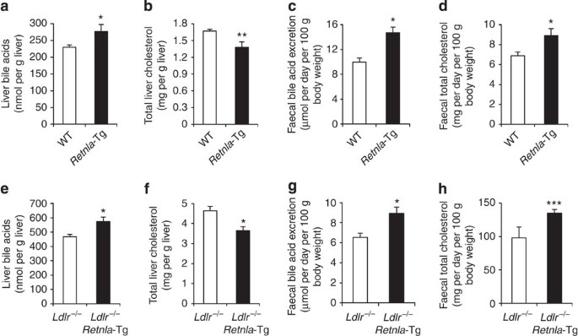Figure 7: Overexpression of Retnla increases hepatic production and faecal excretion of bile acid. (a,b) Levels of (a) bile acid and (b) cholesterol in livers from WT andRetnla-Tg mice fed a HFD for 2 weeks (n=7 for WT mice;n=6 forRetnla-Tg mice). (c,d) Levels of (c) bile acid and (d) cholesterol in the faeces from the same mice as ina,b. (e,f) Levels of (e) bile acid and (f) cholesterol in livers fromLdlr−/−/Retnla-Tg mice andLdlr−/−control littermates fed a HFD for 28 weeks (n=9 forLdlr−/−male mice;n=11 forLdlr−/−/Retnla–Tg male mice). (g,h) Levels of (g) bile acid and (h) cholesterol in faeces from the same mice as ine,f. Data are presented as mean±s.e.m. according to the Mann–WhitneyU-test; *P<0.05; **P<0.01; ***P<0.005. Figure 7: Overexpression of Retnla increases hepatic production and faecal excretion of bile acid. ( a , b ) Levels of ( a ) bile acid and ( b ) cholesterol in livers from WT and Retnla -Tg mice fed a HFD for 2 weeks ( n =7 for WT mice; n =6 for Retnla -Tg mice). ( c , d ) Levels of ( c ) bile acid and ( d ) cholesterol in the faeces from the same mice as in a , b . ( e , f ) Levels of ( e ) bile acid and ( f ) cholesterol in livers from Ldlr −/− / Retnla -Tg mice and Ldlr −/− control littermates fed a HFD for 28 weeks ( n =9 for Ldlr −/− male mice; n =11 for Ldlr −/− / Retnla –Tg male mice). ( g , h ) Levels of ( g ) bile acid and ( h ) cholesterol in faeces from the same mice as in e , f . Data are presented as mean±s.e.m. according to the Mann–Whitney U -test; * P< 0.05; ** P< 0.01; *** P< 0.005. 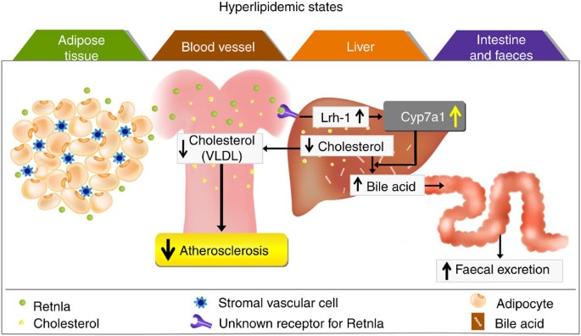Figure 8: Schematic model of the mechanism of the atheroprotective action of Retnla. In states of hyperlipidemia, Retnla production is markedly induced in adipose tissue. Retnla promotes the conversion of cholesterol into bile acid by enhancement of hepatic Cyp7a1 gene transcription through Lrh-1 induction, leading to a subsequent increase in faecal bile acid excretion. The reduction of hepatic cholesterol levels causes a decrease in VLDL cholesterol level in the blood. The reduced blood cholesterol level contributes to the attenuation of atherosclerosis. Full size image Figure 8: Schematic model of the mechanism of the atheroprotective action of Retnla. In states of hyperlipidemia, Retnla production is markedly induced in adipose tissue. Retnla promotes the conversion of cholesterol into bile acid by enhancement of hepatic Cyp7a1 gene transcription through Lrh-1 induction, leading to a subsequent increase in faecal bile acid excretion. The reduction of hepatic cholesterol levels causes a decrease in VLDL cholesterol level in the blood. The reduced blood cholesterol level contributes to the attenuation of atherosclerosis. Full size image We demonstrated that Retnla is an adipokine that exerts favourable effects on hypercholesterolaemia and atherosclerosis by enhancing cholesterol excretion in the form of bile acids. Although previous studies showed that various adipokines have important roles in metabolic diseases [3] , little is known on the role of Retnla in metabolic disease. To our knowledge, ours is the first report to demonstrate the function of Retnla in hypercholesterolaemia and atherosclerosis. Retnla is a resistin family protein, which share cysteine-rich domains at their C-termini. To date, the resistin family is known to include four members: Retnla, Retnlb, resistin and Retnlg [9] . Interestingly, these family members each show unique tissue distribution, raising the possibility of their differential roles in the pathogenesis of diseases. Retnla is expressed mainly by hematopoietic cells and stromal vascular cells but not by adipocytes in WAT [12] , [37] , [43] , [44] . Retnlb is expressed abundantly in the colon in both mouse and human, and expression can also be induced in macrophages under the proper inflammatory conditions [12] , [44] , [45] . In mice, resistin is primarily produced in adipocytes, whereas in humans, resistin is mainly derived from monocytes and macrophages [19] , [46] . Retnlg is expressed abundantly in the colon, lung and spleen [47] . HFD consumption induced secretion of Retnlb, resistin and Retnlg into the serum of C57BL/6J mice [47] , but the HFD-induced secretion of Retnla has not been reported. In this study, we found that Retnla concentrations in serum were increased in HFD-fed C57BL/6J and Ldlr −/− mice, suggesting that Retnla could be related to hyperlipidemia. This result led us to study the function of Retnla in hyperlipidemia in vivo . By generating mice that either lack or overexpress Retnla, we defined a critical role for Retnla in mediating reduction in cholesterol. Retnla overexpression and deficiency did not significantly affect the compensatory expression of other Relm family members in WAT after HFD feeding. Even though Retnla has not been identified in the human genome, human resistin is more similar in expression pattern to mouse Retnla than to mouse resistin, suggesting that the functional role of Retnla may be related to that of human resistin. Resistin, a well-known adipokine, has been implicated in the induction of various metabolic abnormalities, such as obesity [48] , fatty liver disease [49] , hyperlipidemia [50] and atherosclerosis [7] . Although Retnla and resistin belong to the same protein family, our data demonstrate that Retnla and resistin could have opposing actions, even within the rodent. Resistin has been reported to express in both mouse and human, but Retnla has been identified only as mouse gene [9] . Furthermore, Retnla and resistin have differential expression patterns in mouse adipose tissue [12] , [19] . Such differences of Retnla and resistin between mouse and human might explain the possibility for differential roles of these two isoforms. Considering that mice are more resistance to atherosclerosis than humans, Retnla-mediated cholesterol metabolism may be one of underlying mechanisms responsible for murine resistance to atherosclerosis. Therefore, it seems worthwhile to find the functional human counterpart of mouse Retnla for treating human atherosclerosis. Adipokines are mainly secreted from adipocytes and/or macrophages in adipose tissue and have an important role in metabolic diseases, such as type 2 diabetes, dyslipidemia and atherosclerosis [3] . However, nearly every known adipokine has shown disease-promoting actions, with the exception of adiponectin and leptin [3] . Adiponectin −/− mice develop exacerbated diet-induced insulin resistance and augmented atherogenesis when crossed with ApoE −/− mice [51] , [52] , whereas elevated plasma adiponectin caused by adenovirus-mediated gene transfer suppresses the development of atherosclerosis in ApoE −/− mice [8] , [53] . A genetic deficiency of leptin ( ob/ob mice), as well as mutation in the leptin receptor ( db / db mice), also leads to diabetes and obesity, and the administration of leptin reverses these changes and reduces plasma and tissue lipids [54] , [55] . In this study, we demonstrated that Retnla deficiency accelerates atherosclerosis with increasing serum cholesterol level and body weight in Ldlr −/− mice fed a HFD. We also showed that Retnla concentration was higher in ob / ob mice than ob /+ mice. These data suggest that Retnla may be related to hyperlipidemia and obesity, major risk factors of atherosclerosis. Atherosclerosis is an inflammatory disease in whose pathogenesis macrophages play an important role [23] , [38] . Among Relm family members, Retnlb and resistin are implicated as mediators of inflammation [46] , [56] , [57] and abundantly expressed in macrophages of atheroma involved in atherosclerosis development [45] , [58] . Several in vitro and in vivo studies support that Retnlb and resistin are positive regulators in the pathogenesis of atherosclerosis [7] , [45] , [56] , [57] , [58] , [59] , [60] , [61] . Retnlb contributes to atherosclerosis development via induction of lipid accumulation, and upregulation of inflammatory cytokines such as TNF-α, IL-1β and IL-6 (ref. 45 ). Resistin promoted activation of vascular endothelial cells [61] , recruitment of other immune cells [56] and secretion of proinflammatory factors TNF-α and IL-12 in macrophages [57] . Recent work using resistin-overexpressing mice showed that resistin exacerbated atherosclerosis in Ldlr −/− mice [7] . Furthermore, Reilly et al . [62] demonstrated a close correlation between resistin levels and the severity of cardiovascular disease. Thus, it is possible that Retnlb and resistin exert their proatherosclerotic effects by inducing inflammatory responses. Recent work using Retnla −/− mice suggests that physiological and pathophysiological functions of Retnla during inflammatory processes are complex; Retnla has both anti-inflammatory and proinflammatory properties. For example, in a model of dextran sodium sulphate-induced colitis, Retnla deficiency protected against impaired glucose tolerance and colitis [13] , [18] , while in a model of chronic inflammation by Schistosoma mansoni infection, both the lung inflammation and liver fibrosis were increased by Retnla deficiency via an enhanced Th2 immune responses [36] , [37] . These results suggest that the beneficial and detrimental roles of Retnla in inflammatory diseases are likely influenced by the type of immune stimulus, the duration of the stimulus exposure and the tissue type. In this study, we showed that, although there were no significant changes in the expression of M1/M2 genes both in vitro and in vivo , Retnla deficiency caused larger plaques containing more macrophage infiltrations and necrotic area in Ldlr −/− mice. Our results raise the possibility that Retnla may have some roles in chronic inflammatory processes in tissue associated with atherosclerosis such as the aorta. However, further studies are needed to understand the exact function of Retnla in the inflammatory processes of atherosclerosis. Our experiments showed that Retnla -Tg mice have an increased susceptibility to diet-induced hypercholesterolaemia. In particular, there were significant increases in hepatic cholesterol degradation and bile acid production through the upregulation of Cyp7a1 and Cyp8b1 expression in HFD-fed Retnla -Tg mice, leading to reduced serum cholesterol levels and increased faecal bile acid excretion. However, Retnla overexpression did not affect serum cholesterol levels in normolipidemic mice, implying the possibility that the cholesterol-lowering effects of Retnla may be mediated by some factors specifically induced during hyperlipidemia, including farnesoid X receptor, small heterodimer partner, Lrh-1, liver X receptor α and hepatocyte nuclear factor-4α, nuclear receptors that control the expression of Cyp7a1 and/or Cyp8b1 (refs 29 , 63 , 64 , 65 ). In this study, we showed that, among the possible regulating factors, only Lrh-1 expression was unregulated in rRelmα-treated hepatocytes and livers of Retnla -Tg mice. Furthermore, Lrh-1 knockdown significantly reduced Retnla-induced Cyp7a1 expression and transactivation in hepatocytes. These results suggest that Lrh-1 is essential for Retnla-induced Cyp7a1 expression and that the Retnla/Lrh-1/Cyp7a1 signalling pathway has an important role in maintaining cholesterol homeostasis by controlling hepatic cholesterol degradation and bile acid production. However, the specific molecular and cellular mechanisms leading to these effects by Retnla remain to be elucidated. In summary, we identified Retnla as a new atheroprotective adipokine having a cholesterol-lowering effect caused by enhanced cholesterol excretion in the form of bile acids under hyperlipidemic states. Our results using two different rodent models that either overexpress Retnla or lack Retnla provide evidence that Retnla controls the link between cholesterols and atherosclerosis and reveal that Retnla is an attractive novel target for therapeutic intervention for the treatment of hypercholesterolaemia and hypercholesterolaemia-induced atherosclerosis. Generation of Retnla −/− mice The Retnla gene was isolated by PCR from genomic DNA extracted from the liver of C57BL/6J mice. The targeting vector was constructed by replacing all exons (exons 1–4) of the mouse Retnla gene with neomycin-resistance gene cassettes ( neo ) and inserting a herpes simplex virus thymidine kinase driven by the PGK promoter into the genomic fragment for negative selection. After each targeting vector was transfected into ES cells, G418 and ganciclovir double-resistant colonies were selected and screened by PCR. Recombination was further confirmed by Southern blot analysis. Homologous recombinant clones were individually microinjected into blastocysts derived from C57BL/6J mice and transferred to pseudopregnant females. Mating of chimeric male mice with C57BL/6J female mice resulted in the transmission of each mutant allele to the germ line. The resulting Retnla +/− mice were backcrossed to the C57BL/6J background for at least seven generations and then interbred to generate Retnla −/− mice. For the hyperlipidemia and atherosclerosis study, Retnla −/− mice were cross-bred with Ldlr −/− mice generating Ldlr −/− Retnla −/− mice. Retnla genotype status was determined by PCR analysis of tail DNA using the following primers: 5′-GAGCCTGCCAGAGTCTGATACTCAC-3′ (Retnla forward), 5′-GTGTTATCTCCTTTCCTGCCCCC-3′ (Retnla reverse) and 5′-TGTGGCGGACCGCTATCAGGA-3′ (Neo reverse). Ldlr genotype status was also determined by PCR analysis of tail DNA using the following primers: 5′-ACCCCAAGACGTGCTCCCAGGATGA-3′ (Ldlr forward), 5′-CGCAGTGCTCCTCATCTGACTTGT-3′ (Ldlr reverse) and 5′-AGGTGAGATGACAGGAGATC-3′ (Neo reverse). Generation of Retnla -Tg mice Retnla transgenic mice were produced using a pCAGGS expression vector containing a cytomegalovirus enhancer fused to the ubiquitously expressed chicken beta-actin promoter. Mouse Retnla cDNA was obtained by RT–PCR from RNA isolated from the lung and cloned into the Eco RI sites of the pCAGGS vector. The construct was sequenced and introduced into the germ line of C57BL/6J mice by pronuclear injection into a one-cell mouse embryo. Two founders (lines 1800 and 0011) were identified by PCR analysis of tail DNA using the primers 5′-CTCCACTGTAACGAAGACTC-3′ (forward) and 5′-GCAGTGGTCCAGTCAACGA-3′ (reverse). The transgenic mice were bred to be hemizygous for the transgene. Non-transgenic littermates were used as controls. For the hyperlipidemia and atherosclerosis studies, Retnla transgenic mice were cross-bred with Ldlr −/− mice to produce Ldlr −/− / Retnla -Tg double-mutant mice. The Ldlr and Retnla genotype status was determined by PCR analysis of tail DNA. Animal studies and diet For the hyperlipidemia and atherosclerosis studies, mice were switched from a SD to a HFD or HFHC diet at 8 weeks of age and maintained on that diet (Research Diets). The HFD consisted of 0.15% cholesterol and 21% fat and the HFHC diet contained 1.25% cholesterol, 15% fat and 0.5% sodium cholate. The length of HFD or HFHC diet feeding is specified in each figure legend. All mice were given water and food ad libitum and were kept in a room with a light cycle lasting from 07:00 hours to 19:00 hours. All animal studies were conducted in accordance with protocols approved by the IACUC of Ewha Womans University. Fractionation of epididymal WAT Adipocytes and SVF were isolated from epididymal WAT of 8-week-old male C57BL/6J mice as previously described [66] , with minor modifications. In brief, WAT dissected from male mice fed a SD or HFD were minced and digested with 2 mg ml −1 collagenase type I (Roche) in Hank's balanced salt solution (Thermo Scientific) containing 1% BSA at 37 °C for 45 min with gentle shaking. The digested tissues were filtered through a 100-mm filter to remove undigested material and the filtrates were centrifuged at 250 g for 5 min. Floating cells and the pellet were recovered as the mature adipocyte fraction and the SVF, respectively. The resulting cells were washed twice with ice-cold phosphate-buffered saline (PBS) (pH 7.4). Purification of recombinant Retnla protein To isolate intact native Retnla proteins without any trace of the tag (rRelmα), Retnla cDNA was inserted into the Xho 1/ Bam H1 site of the pET-17b vector, and the T7 tag from the cloned pET-17b was removed. The resultant vector allowed the expression of intact native Retnla proteins (amino acids 24–112). After transfection of the pET construct into the BL21 (DE3) strain, protein expression was induced with 0.1 mM IPTG at 25 °C for 6 h. The Retnla protein was predominantly expressed as an inclusion body, and refolding was carried out as previously described [67] , with minor modifications. The cells were suspended in 50 mM Tris–HCl (pH 8.5) containing 1 mM EDTA and 1 mM 4-(2-aminoethyl)benzenesulfonyl fluoride, and disrupted by sonication. After centrifugation, the pellet was washed with buffer containing 0.1% Triton X-100 and 1 mM EDTA, and was resuspended in 20 mM Tris–HCl (pH 8.5), containing 5 mM dithiothreitol, 1 mM EDTA and 8 M urea. After clarification, the soluble fraction was applied to a Q-Sepharose column (Amersham). The denatured protein was refolded by 20-fold dilution with 20 mM Tris–HCl (pH 8.5) containing 1 mM EDTA, 2 mM reduced glutathione and 1 mM oxidized glutathione, and by further incubation for 72 h at 4 °C. After centrifugation, the supernatant was applied to a Q-Sepharose column (Amersham) and the eluted protein was dialyzed against 10 mM Tris–HCl (pH 7.5) containing 25 mM NaCl. Protein concentration was determined by ultrafiltration using Amicon filter (Millipore Corporation). Antibodies For preparation of anti-Retnla antibody, a GST-Retnla fusion protein construct containing an 89-amino acid peptide corresponding to amino acid residues 24–112 of Retnla was prepared by cloning the Eco RI- Xho I fragment of the retnla cDNA in the pGEX-4T1 GST fusion vector and was expressed in the bacterial strain BL21 (DE3). Anti-Retnla polyclonal antibody was raised in rabbit against the GST-Retnla fusion protein and further purified by Affinity chromatography (Young In Frontier, Seoul, Korea). The antibody to apoB100 and apoB48 was purchased from Biodesign International (cat. No. K23300R, rabbit IgG), the antibodies to Moma-2 were obtained from AbD Serotec (cat. No. MCA519G, rat IgG) and GAPDH antibody was from Santa Cruz Biotechnology (cat No. SC-25778, rabbit IgG). Immunofluorescence and histology For immunofluorescence staining, epididymal WATs and hearts were fixed in 10% formalin for 24 h, and embedded in optimal cutting temperature compound for frozen sections. Cryosections of WAT (50 μm) and aortic roots (6 μm) were prepared and stained with primary anti-Retnla (1:50 dilution) and anti-Moma-2 (1:100 dilution) antibody, respectively. After incubation with primary antibody, the sections were incubated with secondary antibody (Alexa Fluor-488 (green) and Alexa Fluor 594 (red); Invitrogen; 1:100 dilution) for 30 min in the dark. 4',6-diamidino-2-phenylindole dihydrochloride staining was employed as a counterstain for fluorescence. Negative control sections were prepared in a similar manner using rabbit IgG or rat IgG isotype control antibody (Santa Cruz Biotechnology). Sections were analysed by confocal microscopy on a Zeiss LSM-510 META Laser Scanning Microscope (Carl Zeiss). For histological examination, aortic root cryosections were stained with Oil red O, hematoxylin and eosin and picrosirius red. Images of sections were digitally photographed and analysed by using AxioVision (Carl Zeiss). Assessment of atherosclerosis Mice were euthanized by CO2 inhalation, and their hearts and aortas were perfused with PBS through the left ventricle. After fixation with 10% formaldehyde overnight, the hearts were embedded in OCT compound for frozen section preparation. The aortas were dissected from the proximal ascending aorta to the bifurcation of the iliac artery, and adventitial fat was removed. For en face analysis, aortas were split longitudinally, pinned onto flat black silicone plates, and fixed in 10% formaldehyde overnight. Aortic root sections and aortas were stained with Oil red O for 4 h, washed with briefly PBS and digitally photographed at a fixed magnification. Total aortic area and lesion area were calculated using AxioVision (Carl Zeiss). Measurement of serum cholesterol Mice were fasted for 4 h after the indicated feeding regimen and were anesthetized using isoflurane for retro-orbital phlebotomy. Serum was prepared by spinning freshly collected blood in a cooled centrifuge at 1500 g for 20 min. The clear supernatant was collected and stored at −80 °C until use. Serum total cholesterol levels were determined using a Hitachi autoanalyzer. For fractionation of lipoproteins, pooled mouse serum (200 μl) was separated by FPLC using a Superose 6HR 10/30 column (Amersham) [68] . Lipoproteins were eluted at a constant flow rate of 0.5 ml min −1 with PBS containing 0.02% EDTA and 0.02% sodium azide. Cholesterol levels of FPLC fractions were measured using enzymatic kits according to the manufacturers’ protocols (Human). Immunoblotting For Retnla detection, protein from the liver tissues was extracted with RIPA buffer (25 mM Tris–HCl, pH 7.6, 150 mM NaCl, 1% NP-40, 1% sodium deoxycholate, 0.1% SDS) containing complete protease inhibitor cocktail (Roche) and adipocytes and SVF isolated from WAT were also lysed in the same buffer. Protein in the amounts of 80, 50 and 30 μg were resolved using 4–20% SDS–PAGE (Roche). Mouse serum was filtered through a 100,000-Dalton cut-off Amicon filter device (Millipore Corporation), and 40 μl was analysed by 4–20% SDS–PAGE. For detection of apoB100 and apoB48, the top fraction of VLDL from FPLC (40 μl) or 4 h-fasted whole serum (1 μl) was separated on 4% denaturing SDS–PAGE, and blots were incubated overnight at 4 °C with the primary antibodies: Retnla (1:2,000 dilution), apoB100 and apoB48 (1:1000 dilution) and glyceraldehyde-3-phosphate dehydrogenase (1:1,000 dilution). HRP-coupled secondary antibody (Millipore Corporation) was used at a 1:5,000 dilution at room temperature for 1 h, followed by detection using the ECL system. Densitometric analyses were carried out using TINA 2.0 software. ELISA Serum Retnla and adiponectin levels were measured with a commercially available RELM-alpha Enzyme Immunoassay kit (RayBiotech) and Adiponectin Duo-set kit (R&D Systems), respectively, according to the manufacturer’s instructions. RNA isolation and qRT–PCR analysis Total RNA from cells and tissues was extracted using the Trizol reagent (5 PRIME). Then, 1.5 μg RNA was quantified spectrophotometrically and reverse transcribed into complementary DNA, using the RevertAid First Strand cDNA Synthesis Kit (Fermentas) according to the manufacturer's instructions. qRT–PCR was performed with a two-step using an ABI Prism 7300 Sequence Detection System (Applied Biosystems) and SYBR Green PCR master mix (KAPA Biosystems). The PCR conditions were as follows: 95 °C for 3 min, followed by 40 cycles of 95 °C for 3 s and 60 °C for 30 s. Relative mRNA expression values were normalized to the level of β-actin expression. Primers designed for amplification are listed in Supplementary Table 2 . Microarray analysis Array processing was conducted using the Affymetrix Mouse Genome 430 2.0 array, following the Affymetrix protocol. To identify differentially expressed transcripts, pairwise comparisons were carried out using GenPlex software (Istech Corporation). qRT–PCR was used to validate results from the microarray results. Cell culture and treatment Murine AML-12 cells were cultured in DMEM/F12 (1:1) medium containing 10% heat-inactivated fetal bovine serum (FBS) (Hyclone) and supplemented with 5 μg ml −1 insulin (WelGENE), 5 μg ml −1 transferrin (WelGENE), 5 μg ml −1 selenium (WelGENE) and 40 ng ml −1 dexamethasone (Sigma). Cells were serum-starved with DMEM/F12 (1:1) containing 0.5% heat-inactivated FBS for 4 h before treatment with or without 100 nM rRelmα. RNA interference and luciferase assays For the siRNA experiment, cells were transfected with 20 nM of siRNA against mouse Lrh-1 (Dharmacon) using Dharma FECT 1 transfection reagent (Dharmacon). Following a 48 h transfection period, cells were treated for 6 h with or without 100 nM rRelmα. For luciferase report assays, the luciferase reporter plasmid, pGL3 basic vector (Promega), carrying a 3.2-kb portion of mouse Cyp7a1 promoter was kindly provided by Professor Hueng-Sik Choi. Cells were first transfected with siRNA for 24 h before being transfected with 0.1 μg of Cyp7a1 luciferase reporter plasmid using Fugene HD (Promega). At 48 h after the second transfection, the cells were treated with or without rRelmα (100 nM), and 6 h later, protein extracts were assessed for luciferase activity (Promega) according to the manufacturer’s instructions. Retnla-binding study rRelmα was labelled with Alexa 488, according to the manufacturer’s instructions (Invitrogen). Before incubation with rRelmα-Alexa 488 (1 μg ml −1 ), the cells were changed into fresh complete media, and then cells and incubation mixtures containing rRelmα–Alexa 488 were pre-cooled on ice for 15 min. Incubation with the fluorescent-conjugated rRelmα was processed for 60 min in AML-12 cells, and then for 30 min in mouse primary hepatocytes. The cells were rinsed in ice-cold PBS, fixed in 4% paraformaldehyde for 10 min and rinsed again three times for 15 min in PBS. 4',6-diamidino-2-phenylindole dihydrochloride stain was employed to counterstain for fluorescence. After washing in PBS, coverslips were mounted onto glass slides using Vectashield mounting media (Vector). Images were analysed using LSM Image Examiner (Carl Zeiss, German). Isolation and culture of peritoneal macrophage Peritoneal macrophages were isolated from 8-week-old Retnla −/− and WT male mice by peritoneal lavage with 10 ml of ice-cold PBS and were plated in RPMI-1640 medium (Invitrogen) containing 10% heat-inactivated FBS (Hyclone). After a 3–4 h incubation at 37 °C and 5% CO 2 , non-adherent cells were removed, leaving adherent cells for use in the experiments. To promote differentiation into M1 or M2 macrophages, the cells were stimulated with 100 ng ml −1 lipopolysaccharide (LPS; Sigma) or 10 ng ml −1 IL-4 (R&D Systems), respectively, for 24 h. Hepatic and faecal cholesterol content For the analysis of hepatic cholesterol, aliquots of liver samples (150 mg) were homogenized in two volumes of homogenization buffer (50 mM Tris–HCl, pH 7.4, 154 mM KCl, 1 mM EDTA). The homogenate was centrifuged at 15,000 g for 3 h at 4 °C. The cholesterol concentration in the supernatant was assayed using enzymatic kits according to the manufacturers’ specifications (Human). For analysis of faecal cholesterol, faeces from individually housed mice were collected, weighted and freeze-dried for 24 h. Then the faeces were ground to a fine powder and 0.1 g of the powdered faeces was used to extract cholesterol according to the modified method of Folch et al . [69] The faeces were homogenized in 2.5 ml of 0.9% NaCl solution and incubated with 5 ml of chloroform–methanol (2:1) at 4 °C with constant agitation. After overnight incubation, the samples were centrifuged at 2,000 g for 20 min at 4 °C. The lower chloroform phase was then removed, transferred to a new tube and dried under N 2 gas. Samples were then resuspended in chloroform–Triton X-100 (1%) solution, dried under N 2 gas and finally, resuspended in water. The quantities of total cholesterol in the faecal extracts were assayed as above. Bile acid analysis Measurement of faecal and tissue bile acids was performed as reported previously [70] . Faecal powder (0.1 g) was added to 10 ml of 75% ethanol. The bile acid pool size was determined by measuring the total amount of bile acid in the liver, gallbladder and small intestine. These tissues were homogenized together in 25 ml of 75% ethanol. The faeces and tissue homogenates were incubated at 50 °C for 2 h to extract bile acids and centrifuged at 2,000 g for 30 min. For the assay, the supernatant was diluted 1:4 in 25% PBS solution. Serum samples were used immediately. Bile acids were measured enzymatically using the total bile acid colorimetric assay kit according to the manufacturer's instructions (Bio-Quant). Statistical analyses Results are expressed as the mean±s.e. Differences between the two animal groups were assessed using a two-tailed non-parametric Mann–Whitney U -test. The unpaired two-tailed Student’s t -test was used to evaluate results from the in vitro study. Microarray data were analysed by one-way analysis of variance. The means of the two groups were considered significantly different when P <0.05. How to cite this article : Lee, M.-R. et al . The adipokine Retnla modulates cholesterol homeostasis in hyperlipidemic mice. Nat. Commun. 5:4410 doi: 10.1038/ncomms5410 (2014). Accession codes : Microarray data have been deposited at the Gene Expression Omnibus (GEO) under the accession code GSE58214 .